On the absence of intrahelical DNA dynamics on the μs to ms timescale DNA helices display a rich tapestry of motion on both short (<100 ns) and long (>1 ms) timescales. However, with the exception of mismatched or damaged DNA, experimental measures indicate that motions in the 1 μs to 1 ms range are effectively absent, which is often attributed to difficulties in measuring motions in this time range. We hypothesized that these motions have not been measured because there is effectively no motion on this timescale, as this provides a means to distinguish faithful Watson–Crick base-paired DNA from damaged DNA. The absence of motion on this timescale would present a ‘static’ DNA sequence-specific structure that matches the encounter timescales of proteins, thereby facilitating recognition. Here we report long-timescale (~10–44 μs) molecular dynamics simulations of a B-DNA duplex structure that addresses this hypothesis using both an ‘Anton’ machine and large ensembles of AMBER GPU simulations. Beyond the familiar and characteristic structure of the DNA Watson–Crick (WC) double helix [1] , the differential dynamics and deformability of DNA are very important for its biological functions. At the macroscale, torsional stress and supercoiling play key roles in many of the functions of DNA ranging from transcription and packing in the chromosome to DNA replication and its regulation [2] , [3] . Likewise, at the microscale and on the level of individual base pairs, DNA breathing, bending, twisting, groove fluctuations and base pair opening are critical for function and important for recognition processes [4] , [5] . Many different experimental approaches have been applied to give insight into DNA dynamics, which can be separated into measurements on very fast timescales (less than 100 ns) to those probing slower events—such as internal base pair opening—on timescales of milliseconds and longer. On the fast timescales, many different experiments probe specific indicators of motion, such as particular pair interactions or site interactions that can be uncovered by the applied instrument. Characteristic vibrations and/or interactions can be probed and exposed on femtosecond to nanosecond timescales with Fourier transform infrared difference spectroscopy [6] , two-dimensional infrared spectroscopy [7] , nonlinear ultrafast vibrational spectroscopy [8] , triplet anisotropy decay [9] , [10] , field cycling NMR methods [11] , as well as electron paramagnetic resonance and pulsed electron–electron double resonance measurements of active nitroxide or other spin labels [12] , [13] , [14] , [15] . All of these methods expose identifiable signals of motion at particular and specific timescales in the femtosecond to nanosecond regime. For example, time-resolved electron emission spectroscopy monitoring the dye Hoechst 33258 bound to DNA shows components of DNA relaxation at 40 ps and 12.3 ns (ref. 16 ), while solution NMR studies of polyadenine tracts showed enhanced sugar puckering and backbone transitions at the junctions on the ps–ns timescale [17] . In contrast, there are other experimental measures that provide a more general picture of the motions on the fast timescale—dynamics that are collectively averaged over all the motions of the DNA, solvent and ions. For example, time-resolved Stokes shifts of dyes bound to duplex DNA display a rich power law behaviour in the fast timescale motions, interpreted from femtoseconds to ~40 ns, with motions that cannot be easily decomposed into subsets of motions on particular timescales [18] , [19] , [20] . Essentially, all of the different experimental approaches paint a consistent picture that suggests a rich and dynamic environment of DNA motions on the fast timescale across the entire fs–ns timescale, a picture that is supported by molecular dynamics (MD) simulations on nanosecond timescales [21] , [22] . Considering timescales longer than 1 ms, the most accurate probes of DNA dynamics and flexibility are likely from NMR spectroscopy [5] . Internal base pair opening of WC paired bases, as inferred from measured imino proton exchange in NMR experiments, is estimated to be on the order of ~5 ms or longer, with open-state lifetimes in the ~100 ns range (refs 23 , 24 , 25 ). Exceptions to this are slightly faster internal base pair opening rates with isolated A–T base pairs (not in A-tracts) [26] and also in d(CG) n repeats [27] , however still with opening rates greater than ~1 ms. Taken together, the experimental investigations suggest rich dynamics within DNA duplexes on timescales faster than a few hundred nanoseconds in terms of bending, twisting, backbone dynamics and sugar puckering, followed on longer timescales by significant dynamics due to internal base pair opening at milliseconds and beyond. Interpretation of the experimental data suggests that there is a gap in the dynamics of WC base-paired DNA on timescales from ~1–5 μs to ~1 ms. Is this gap real or does it appear as a result of the difficulty in measuring dynamics on this timescale? There are three indirect pieces of evidence that suggest that the gap in dynamics is real and also likely to be important for recognition: specialized NMR measurements [28] , [29] , differential scanning calorimetric (DSC) thermodynamic measurements [30] and MD simulations. MD simulations can accurately probe nucleic acid structure and dynamics [21] . However, unlike proteins which have been simulated to the millisecond timescale [31] , the longest published simulations of DNA duplexes are on the 1–4 μs timescale [32] , [33] , [34] . Although many of the properties of the internal helix are converged on the 250–300 ns timescale, the data are not fully converged and longer simulations are necessary to completely relax or sample the backbone conformational sub-states (such as B I /B II , α/γ, sugar puckers), ion distributions and bimodal twist distributions at particular base pair steps. In addition, as terminal base pair opening occurs on a microsecond timescale and can occur in multiple ways, for example, with opening into the major or minor groove, clearly the ‘end-effects’ will not be converged. To understand the dynamics of DNA and convergence in the structural properties on the microsecond timescale, a relatively long ~44 μs MD simulation (ANTON) was run using the special purpose ‘Anton’ MD engine. The DNA is an 18-mer with the sequence d( GCACGAACGAACGAACGC ), hereafter referred to as GAAC, which is one of the sequences used by the ABC consortium to study sequence-dependent DNA structure and dynamics in all tetra-nucleotide repeats [35] , [36] , [37] . Since the initial results observed in the Anton runs were unexpected, with an effective absence of motion beyond the 1–5 μs timescales, an additional ensemble (ENS) set of simulations were performed using the GPU MD engine in AMBER. Specifically, 100 independent MD simulations were run using the standard AMBER force field for DNA at the time (ff99SB with parmbsc0 or equivalently ff12) (refs 38 , 39 , 40 ) on the order of ~900 ns, each with different initial ion placements, leading to an ~80+ μs aggregate MD trajectory. Moreover, to determine if convergence in the dynamics of the internal portion of the helix is also observed in simulations with a completely different nucleic acid force field, an additional set of ensemble simulations was performed with the CHARMM all36 (C36) force field [41] . The results suggest that MD simulations can reproducibly converge the structure and dynamics of the internal portion of a DNA helix. Combined with interpretations from experiment, the MD simulations support the assertion that the gap in WC base-paired DNA helix dynamics from 1 μs to 1 ms is real. Evidence for a gap in the dynamics on the μs-ms timescale There are three indirect pieces of evidence that suggest that the gap in dynamics from the microsecond to the millisecond range in duplex DNA is real and also likely to be important for recognition: specialized NMR measurements, DSC thermodynamic measurements and MD simulations. From NMR experiments, measures of the exchange kinetics of imino protons from resonance line widths and selective longitudinal relaxation times indicate that when a G–T mismatch is present in a duplex, base pair opening times occurred faster than 1 ms (ref. 29 ). More recently, by applying selective off-resonance carbon R 1ρ NMR relaxation dispersion spectroscopy, Al-Hashimi and coworkers [28] were able to more clearly resolve exchange processes of a 1,N6-ethenoadenine (eA) lesion/mismatch in a DNA duplex with timescales on the order of 26±8 μs. Similar NMR experiments on native WC base-paired duplexes without mismatches or lesions are not able to resolve any exchange processes faster than 1 ms—with the exception of terminal base pair fraying, which occurs on the microsecond timescale [42] , [43] , [44] . Similarly, thermodynamic signatures from DNA damage are clearly evident in DSC experiments that are likely to impact the dynamics and which are not seen in undamaged DNA [30] . MD simulations of the GAAC 18-mer duplex To better understand the convergence of the structure and dynamics of a B-DNA duplex in MD simulations and reproducibility of independent simulations, a variety of MD simulations were performed on the ‘Anton’ MD engine and also with AMBER. 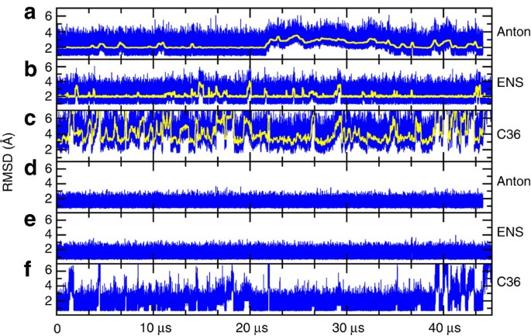Figure 1: RMSD of the frames sampled in MD simulations to time-averaged reference structures. Shown in the top three panels are RMSD values over all atoms (yaxis in Å) in blue and running averages over 5,000 frames in yellow for the Anton simulation (a), the ENS simulations (b) and the CHARMM C36 simulations (c). In the bottom three panels are the RMSD values omitting the four terminal base pairs on each end for Anton (d), ENS (e) and CHARMM C36 (f). Whereas the AMBER ff12 data is flat due to no significant base pair opening beyond the first two to three base pairs, the C36 data still shows excursions away from lower RMSD values due to more significant perturbation from base pair fraying on the ends of the helix. The reference structure for the Anton and ENS simulations is an average structure calculated over 10 μs from an initial independent Anton simulation with ff12. The reference structure for the C36 simulations is an average structure calculated over the first 10 μs of the C36 ENS runs. When calculating the average structure, frames were RMS fit to the first frame. Figure 1 displays the root mean square deviation (RMSD), or overall similarity of each trajectory to a reasonably converged reference structure as a function of time, with lower RMSD indicating greater similarity. For the AMBER Anton and ENS simulations, the reference is the average structure over 10 μs from an additional independent Anton run. Since the C36 runs had larger fluctuations compared with the other two, its reference is the average structure over the first 10 μs of the aggregate C36 runs. Overall, the structures sampled in the MD simulations remained close to their respective reference structures on the 10–40 μs timescale. The RMSD values fluctuate between 1 and 6 Å (or up to ~8 Å with C36), noting that the transient larger deviations (seen as peaks or bumps in the running average plot) are due to terminal base pair opening events ( Fig. 1a–c ). Such events can occur on either one end of the duplex or on both sides simultaneously and are complex molecular processes. For example, the base pairs can partially open, open completely into the minor or major groove and may open multiple base pairs. In each of the simulations, multiple short-lived terminal base pair opening events are present, with significantly faster terminal base pair opening and larger excursions from the reference structure evident with the C36 force field. As the opening events are complex, it is clear that insufficient events are observed to demonstrate convergence on the timescale of these simulations. The RMSD plot for the longer Anton simulation ( Fig. 1a ) shows a long-lasting deviation that represents base flipping into the minor groove followed by an opening of the second base pair as well. The event starts at ~21.5 μs and by the end of the simulation, the two opened base pairs completely reform their WC base pairing. The RMSD plot for the AMBER ENS simulations ( Fig. 1b ) does not show such large deviations mainly due to the shorter duration of the individual MD trajectories, which have less of a chance to find and sustain a terminal base pair opening event. Figure 1: RMSD of the frames sampled in MD simulations to time-averaged reference structures. Shown in the top three panels are RMSD values over all atoms ( y axis in Å) in blue and running averages over 5,000 frames in yellow for the Anton simulation ( a ), the ENS simulations ( b ) and the CHARMM C36 simulations ( c ). In the bottom three panels are the RMSD values omitting the four terminal base pairs on each end for Anton ( d ), ENS ( e ) and CHARMM C36 ( f ). Whereas the AMBER ff12 data is flat due to no significant base pair opening beyond the first two to three base pairs, the C36 data still shows excursions away from lower RMSD values due to more significant perturbation from base pair fraying on the ends of the helix. The reference structure for the Anton and ENS simulations is an average structure calculated over 10 μs from an initial independent Anton simulation with ff12. The reference structure for the C36 simulations is an average structure calculated over the first 10 μs of the C36 ENS runs. When calculating the average structure, frames were RMS fit to the first frame. Full size image Although the traditional RMSD plots suggest that the MD sampled structures remain near the reference structure, particularly when the terminal base pairs are omitted ( Fig. 1d–f ), they do not directly imply stability or provide insight into ‘convergence’ of the MD simulations. Convergence, in this context, means effectively a complete sampling of conformational events observed over particular timescales. A simple way to visualize this is by comparison of the time-averaged structures calculated over different regions of the MD trajectory. When this is done for MD structures on 1–5 μs timescales from the initial Anton MD trajectories, we were very surprised to find that average structures compared over different microsecond time intervals were nearly identical. Given that DNA is known to be dynamic, with characteristic bending, twisting and breathing motions, the absence of motion on the microsecond timescale—despite a dearth of experimental measures of dynamics on this timescale with the exception of terminal base pair fraying—initially caused us concern. Given that the Anton machine is known to make approximations for speed, we initially hypothesized that the effective lack of motion may be due to either Anton or alternatively artifacts of the applied force field. This caused us to reproduce MD trajectories independently using AMBER on GPUs and CPUs, and also—thanks to access to large-scale GPU resources on XSEDE KIDS/Keeneland and the Blue Waters Petascale Resource—to perform ensembles of independent MD runs with both the AMBER ff12 and CHARMM C36 force fields. Convergence of the DNA structure over time Shown in Fig. 2 are molecular graphics representations of the representative structures (those closest to their cluster centroid) from 10 clusters generated by clustering the MD trajectories based on structural similarity after smoothing over different time intervals (specifically 50 ns, 325 ns, 2 μs and 8 μs) with CPPTRAJ [45] . The terminal base pairs on each end were not used during the clustering. The 10 representative 50 ns averaged structures show that even at this short timescale, the motions of the bases on the internal portions of the helix are fairly well converged with structural deviations, or differences, most evident on the backbone and in the termini. By 325 ns of time averaging, the internal helix is even more converged or overlapping, with the most significant structural differences occurring on the termini. By 2 μs of time averaging, the 10 overlapping structures are extremely close to each other, with only small differences observed at the termini. By 8 μs of time averaging, there is a near-complete overlap of the structures with only very small deviations at the termini. 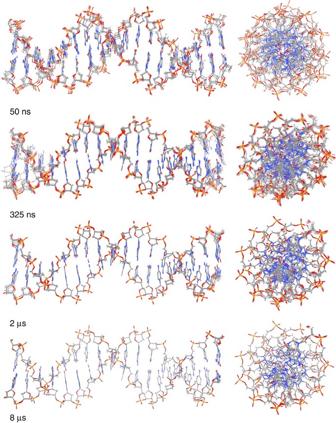Figure 2: Structures from time-averaged or smoothed MD trajectories. Straight coordinate running averages over different time windows (50 ns, 325 ns, 2 μs and 8 μs) of RMS fit snapshots at 50 ps intervals were calculated for the AMBER ENS MD simulations and the resulting trajectories were clustered into 10 clusters (using pairwise RMSD calculations over all atoms omitting the terminal base pairs from the clustering). The 10 most representative structures (that is, those closest to the centroid of each cluster) are displayed as molecular graphics. Figure 2: Structures from time-averaged or smoothed MD trajectories. Straight coordinate running averages over different time windows (50 ns, 325 ns, 2 μs and 8 μs) of RMS fit snapshots at 50 ps intervals were calculated for the AMBER ENS MD simulations and the resulting trajectories were clustered into 10 clusters (using pairwise RMSD calculations over all atoms omitting the terminal base pairs from the clustering). The 10 most representative structures (that is, those closest to the centroid of each cluster) are displayed as molecular graphics. Full size image As an additional metric to explore convergence, we also applied our previously developed method for calculating the RMSD average correlation (RAC), which shows how the similarity of structures within a trajectory changes when averaged over increasing time windows. The faster the RAC decays, the more rapidly the behaviour of the system approaches the overall average. This is shown in Fig. 3 for each of the simulations using only the heavy atoms of the 10 central base pairs d( GAACGAACGA ) using the same reference structure (the 10-μs average structure from the initial Anton simulation). The decay of the RAC values is extremely fast, such that on the timescale of ~80–130 ns the average RMSD values are already less than 0.1 Å for the AMBER simulations. The decay of the RAC with the ff12 force field continues as the simulation progresses and the average RMSD values plateau. The fast decay suggests a rapid convergence of the dynamics and fluctuations of the central base pairs such that when the averaging occurs over the 1–5 μs timescale, essentially the structure is converged and all the dynamics are absent. This agrees with the previously discussed experimental evidence suggesting a gap in DNA dynamics on the 1 μs to 1 ms timescale. Considering the RAC analysis, the slope is essentially flat by 2.5–5 μs for all of the systems with deviations of less than 0.05 Å by 2 μs for the simulations with the AMBER ff12 force field. In terms of atomic positional fluctuations of the atoms around the average reference structure, by 1 μs of time averaging, the base atom fluctuations are already less than 0.1 Å and the phosphate and sugar atom fluctuations are less than 0.15 Å. With the CHARMM C36 force field, the convergence is slightly slower due to structural distortions induced by the frequent base pair opening which traverses deeper into the helix. This is clearly evident in Fig. 1 in the bottom panel for the C36 simulation, which shows large RMSD fluctuations away from the reference even when the terminal four base pairs on each end are omitted. Despite this, average RMSD values are still less than 0.075 Å by 2.5 μs. These are very small deviations in the structure. Together, the MD simulations suggest that no significant structural changes are to be expected in the central regions of the DNA beyond ~1 μs unless an internal base pair opening event occurs, which as previously mentioned is expected at time ranges between 5 and 100 ms. The inset plot shows the RAC decay at shorter timescales and suggests, interestingly, that the dynamics decay initially faster with the CHARMM C36 force field and then slow; again, this is likely due to the disruption in the internal helix structure resulting from the larger and more frequent terminal base pair opening events. Despite subtle differences, it is clear with either force field that the decay in the RAC is very rapid, with deviations of less than 1 Å already within 10 ns of MD simulation. Given the computational cost of these calculations and expiration of our allocation of computer time on Anton, we do not yet have the results of MD simulations with mismatches. However, further ensemble simulations are underway on the Blue Waters Petascale Resource and various XSEDE resources with faster GPU nodes to explore mismatches and ideally dynamic events from internal base pair opening on the low μs timescale. In addition, although the observed converged average structures with both force fields show general agreement with sequence-specific structural trends expected from experiment [35] , [36] , [37] , [46] , there is no direct way to compare this structure, chosen initially because of its bimodal twist distribution at the central CpG step observed in the original ABC experiments [35] , [36] , [37] , to experiment as an NMR solution structure has not been published. Details on the structure and observed differences with different force fields are discussed in greater detail in subsequent work. 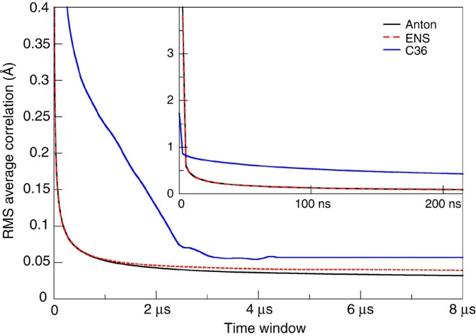Figure 3: Decay in the average RMSD values as the window for time averaging increases. Shown is the RAC for the Anton (solid black line), AMBER ENS (dashed red line) and CHARMM C36 ENS (solid blue line) simulations based on the heavy atoms of the DNA omitting the four terminal base pairs on each end of the helix (that is, using only the 10 central base pairs). Given that the two force fields do not converge to the same average structure, to approach low values in the RAC analysis, the reference structure for the ff12 runs was the 0–10 μs average structure from the initial Anton simulation, while that for the C36 ensemble was the 0–10 μs average structure from the C36 ENS simulations. The inset plot shows the same information, focusing on the initial decay of the average RMSD values over shorter time windows. Figure 3: Decay in the average RMSD values as the window for time averaging increases. Shown is the RAC for the Anton (solid black line), AMBER ENS (dashed red line) and CHARMM C36 ENS (solid blue line) simulations based on the heavy atoms of the DNA omitting the four terminal base pairs on each end of the helix (that is, using only the 10 central base pairs). Given that the two force fields do not converge to the same average structure, to approach low values in the RAC analysis, the reference structure for the ff12 runs was the 0–10 μs average structure from the initial Anton simulation, while that for the C36 ensemble was the 0–10 μs average structure from the C36 ENS simulations. The inset plot shows the same information, focusing on the initial decay of the average RMSD values over shorter time windows. Full size image Convergence and reproducibility of the MD simulations Principal component (PC) analysis can be used to reveal the dominant modes of motion in a trajectory, and comparing PC projections between different MD simulations can provide a metric of similarity between the dominant modes of motion sampled by the different MD trajectories [47] , [48] . To measure how well the motions (that is, the dynamic properties) of DNA in the Anton and ENS simulations converge with respect to each other, we performed PC analysis using both trajectories. 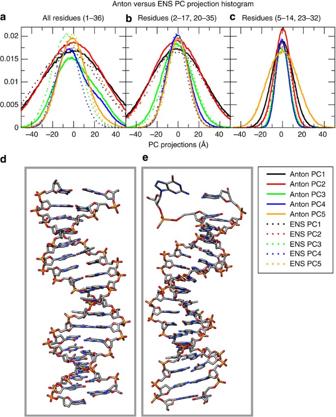Figure 4: Overlap of the independent PC projection histograms from each of the MD simulations from PCs calculated in Cartesian space from the combined Anton and ENS MD trajectories over all DNA atoms. Plot (a) includes all base pairs. Visual inspection shows significant divergence in the histogram overlap of the third (green) and fourth PC (blue). As the terminal base pairs are removed from the analysis (b) and (c), the PC histograms more clearly overlap and sample the same space. The molecular graphics in (d) and (e) are representative structures obtained from the projected frames of the third and fourth PC mode respectively, which show conformational difference due to terminal base pair opening events. Figure 4 shows the overlap of histograms of the PC projections for the five most dominant models of motion from the Anton and ENS simulations (shown as solid and dashed lines respectively). Figure 4a shows the results of the PCA performed on all base pairs. While there is some overlap between the first, second and fifth PCs (corresponding to global DNA bending/twisting motions), there is significantly less overlap for the third and fouth PCs, which happen to correspond to terminal base pair opening events. The Anton simulations have wider distributions for these PCs, indicating these motions are less prevalent in the ENS simulations, which is consistent with the observations of the RMSD plots ( Fig. 1 ) and the fact that the ENS MD simulations are each individually shorter in duration. If the first and last base pairs are removed from the analysis, we notice an overall better overlap between the PCs of both simulations ( Fig. 4b ). If only the central 10 base pairs are included in the analysis ( Fig. 4c ), the histograms are essentially identical. These results suggest that overall the same types of motion are sampled in the two independent simulations, but also that terminal base pair opening events are enhanced in the longer timescale Anton simulation. Figure 4: Overlap of the independent PC projection histograms from each of the MD simulations from PCs calculated in Cartesian space from the combined Anton and ENS MD trajectories over all DNA atoms. Plot ( a ) includes all base pairs. Visual inspection shows significant divergence in the histogram overlap of the third (green) and fourth PC (blue). As the terminal base pairs are removed from the analysis ( b ) and ( c ), the PC histograms more clearly overlap and sample the same space. The molecular graphics in ( d ) and ( e ) are representative structures obtained from the projected frames of the third and fourth PC mode respectively, which show conformational difference due to terminal base pair opening events. Full size image Rapid fluctuations in the groove width Another measurement of interest is groove width, as the space in the grooves is critically important for drug and protein binding. 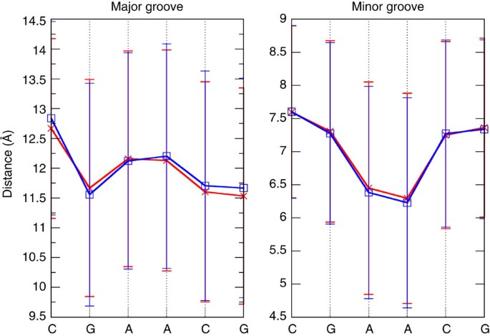Figure 5: Average and s.d. of major and minor groove widths for the ENS (blue lines) and Anton (red lines) simulations. The widths for the central 5′- CGAACG -3′ portion of the helix (residues 8–13, 24–29) are shown. Data was calculated for each frame from the MD trajectory at 50 ps intervals using the Curves+ programme. Figure 5 shows the average and s.d. of the major and minor groove widths for the Anton and ENS simulations. In general, the difference in groove widths between the Anton and ENS simulations are very small, on the order of 0.05 Å (noting that the two terminal base pairs have been omitted from the calculation), and only moderately higher at A15 and C16 with values of ~0.10 and ~0.20 Å for the major and minor groove, respectively, which is due to the Anton long-lived base pair opening event at that end of the helix. Although the distribution of the groove widths are well converged between the two simulations, the s.d. in the groove widths themselves across each simulation are quite large, on the order of ~1.5–1.9 Å. The observed fluctuations in groove width are considerably larger than the sequence-specific structural differences. The MD simulations show that on very rapid timescales, a wide variety of groove widths are sampled, which then effectively converge to the average groove widths on timescales on the order of μs. This corresponds to the timescale for protein or ligand association with the DNA and likely is important for recognition. With the dynamics effectively averaged out in the internal DNA helix on the 1 μs to 1 ms timescale, potential ligands effectively see a consistent structure and can bind by conformational selection (as opposed to induced fit). This contrasts with DNA mismatches or lesions, as discussed previously, which alters DNA dynamics to signal an unusual ‘beacon’ of motions on the μs timescale that may help DNA repair protein recognition. Moreover, as internal base pair opening events occur on much longer timescales (>1 ms) with rapid base pair closing, induced fit by the protein or ligand binding are likely the operational mechanisms for recognition of open states and/or to induce kinking and/or bending. These results, taken together with the current experimental understanding of DNA dynamics, suggest that this gap in DNA dynamics from 1 μs to 1 ms may provide a means for fidelity in recognition. Figure 5: Average and s.d. of major and minor groove widths for the ENS (blue lines) and Anton (red lines) simulations. The widths for the central 5′- CGAACG -3′ portion of the helix (residues 8–13, 24–29) are shown. Data was calculated for each frame from the MD trajectory at 50 ps intervals using the Curves+ programme. Full size image The results of this work suggest that MD simulations can converge the structure and dynamics of the internal portion of a DNA helix and demonstrate reproducibility from independent simulations. The results clearly show fast decay in the dynamics of the DNA helix with both the latest AMBER and CHARMM nucleic acid force fields, and that a large ensemble of independent simulations compared to a single long Anton MD simulation give equivalent results in terms of structure and dynamics, at least for internal base pairs. Motions faster than μs in WC base-paired B-DNA include sampling of different backbone conformational states, rapid fluctuations in the groove widths, sugar repuckering, bending, twisting and sampling of a wide variety of helicoidal parameter distributions, and terminal base pair opening. On the μs timescale, with the exception of terminal base pair fraying, all these motions are effectively averaged out. In the absence of mismatches or lesions in the DNA helix (and with the exception of terminal base pair fraying) other motions are not expected until the ms timescale and this motion will largely be internal base pair opening. The results from MD simulation combined with interpretations from experiment support the assertion that the gap in WC base-paired DNA helix dynamics from 1 μs to 1 ms is real. The B-DNA sequence d( GCACGAACGAACGAACGC ) was generated following the original ABC protocol [35] , [36] , [37] . Simulations were run using the Amber ff99SB (refs 38 , 39 ) force field using the parmbsc0 modifications [40] , the SPC/E water model [49] , neutralizing charge with K + and an excess of K + and Cl − to reach a ~150 m M concentration (that is, an additional 60 ions of each type) with the Dang ion parameters [50] . The initial ion positions were randomized by swapping with a random water molecule such that no ion was closer than 4 Å to any other like ion, and such that all ions were at least 6 Å from the DNA structure. The simulation protocol applied is equivalent to the earlier ABC simulations. Production runs with AMBER were performed at 300 K with weak coupling algorithm for temperature and pressure control (5 ps relaxation time). Long-range interactions were calculated using PME using default settings, SHAKE on bonds to hydrogen and a 2-fs integration time step. For the Anton simulation, the coordinates were recorded every 50 ps using the specialized MD engine Anton, built by DE Shaw Research, Inc. that has been loaned to the Pittsburgh Supercomputing Center. Allocations of computer time on Anton were made available through a competitive proposal and allocation process to researchers in the United States. This process was administered by the Pittsburgh Supercomputing Center and a National Academies Review Committee. The Anton simulations were performed through two allocations of computer time on Anton, each for 1 week on the 512 computing element machine in 2011 and 2012. The total Anton simulation time for the longer simulation was of 44.06 μs. In addition, an earlier initial simulation on Anton was run for over 10 μs. Multiple different versions of the Anton software and microcode (initially 2.4.1 and then 2.4.5) were applied and the available ‘amber_topNrst2cms.py’ script on anton.psc.edu was used with Desmond to convert AMBER parameter and topology inputs into a format appropriate for Anton. During error checking, we noticed that with the parmbsc0 force field C5′, atoms were erroneously specified with a zero mass which was fixed. The Anton supplied ‘guess_chem’, ‘refinesigma’ and ‘subboxer’ programs set up the system and then production runs were initiated at constant 300 K temperature and 1 bar pressure with weak coupling using a coupling time ‘tau’ of 10.0, a maximum and minimum velocity scaling of 1.2 and 0.85 and a maximum and minimum expansion per step of 1.05 and 0.97 and kappa of 4.5 × 10 −5 were imposed. The ‘max_strain’ was set to 0.08 and a 2-fs integration time step with RESPA on the long-range non-bonded interactions every third step was performed. The resulting Anton trajectories were converted to DCD trajectory format using VMD. The ENS (ensemble) simulations were generated using 100 independent simulations starting from the same structure but with randomized ion positions. Each AMBER ff12 simulation was run for no less than 300 ns using either the AMBER12 or AMBER14 PMEMD.cuda [51] , [52] , [53] , [54] , [55] version on either the XSEDE Keeneland or KIDS GPU cluster from Georgia Tech/NICS. The initial 100 ns of MD simulation from each trajectory were deleted to remove any artifacts from equilibration and the remaining frames were concatenated together, resulting in one large 22+ μs trajectory. Given that the dynamics converge so rapidly, the arbitrary choice of 100 ns for omission appears justified. Given queue waits, this required approximately 7 months on nVIDIA M2090 GPUs. While this article was in review, the initial 300 ns trajectories were extended to over ~900 ns per independent run on the Blue Waters Petascale Resource leading to an aggregate trajectory of 80+ trajectory; the extension of these trajectories did not alter any of the results significantly, except for better, albeit not converged, sampling of the terminal base pair opening events. To determine if the gaps in the dynamics of the internal portion of the helix are also observed in simulations with a completely different nucleic acid force field, an additional set of ensemble simulations was performed with the CHARMM all36 (C36) force field [41] . The 100 independent runs on at least the 900-ns timescale were performed with the CHARMM C36 force field, built in an equivalent manner using the CHARMM C36 force field, but with CHARMM TIP3P and ion parameters instead. The files were built using CHARMM version c37b2 after the force fields were converted over to AMBER/PDB/standard DNA naming conventions, and then converted into AMBER compatible input coordinate and parameter/topology formats with the chamber utility of AmberTools. The C36 runs were performed on the NCSA Blue Waters resource. Thanks to access to faster nVIDIA K20 GPUs on Blue Waters, improvements in the performance of the AMBER GPU code, and shorter queue waits, this longer set of trajectories only required two months to generate. All the analysis was performed using a development version of CPPTRAJ [45] and this code is now freely available in the released version of Amber 14. To create average structures as references, the coordinates from the MD trajectories at 50 ps intervals were RMS fit to the first frame over all DNA atoms and a straight coordinate average over the specified interval was performed. Clustering by RMSD was done using the average-linkage algorithm on the MD trajectories at 50 ps intervals using a sieve of 250 frames. DNA structural analysis was made using PTRAJ, CPPTRAJ and Curves+ (ref. 56 ). All the analysis commands, inputs, raw and derived simulation data are available for download at http://www.amber.utah.edu/DNA-dynamics/GAAC . How to cite this article: Galindo-Murillo, R. et al . On the absence of intrahelical DNA dynamics on the μs to ms timescale. Nat. Commun. 5:5152 doi: 10.1038/ncomms6152 (2014).